Internalization and vacuolar targeting of the brassinosteroid hormone receptor BRI1 are regulated by ubiquitination Brassinosteroids are plant steroid hormones that control many aspects of plant growth and development, and are perceived at the cell surface by the plasma membrane-localized receptor kinase BRI1. Here we show that BRI1 is post-translationally modified by K63 polyubiquitin chains in vivo . Using both artificial ubiquitination of BRI1 and generation of an ubiquitination-defective BRI1 mutant form, we demonstrate that ubiquitination promotes BRI1 internalization from the cell surface and is essential for its recognition at the trans -Golgi network/early endosomes (TGN/EE) for vacuolar targeting. Finally, we demonstrate that the control of BRI1 protein dynamics by ubiquitination is an important control mechanism for brassinosteroid responses in plants. Altogether, our results identify ubiquitination and K63-linked polyubiquitin chain formation as a dual targeting signal for BRI1 internalization and sorting along the endocytic pathway, and highlight its role in hormonally controlled plant development. Brassinosteroids (BRs) are polyhydroxylated steroid hormones that regulate plant growth and development [1] . Studies of mutants with defects in BR biosynthesis or signalling demonstrated that BRs play essential roles in nearly all phases of plant development, as these mutants show multiple developmental defects, such as reduced seed germination, extreme dwarfism, photomorphogenesis in the dark, altered distribution of stomata, delayed flowering and male sterility [1] , [2] . BRs are perceived at the cell surface by the membrane-bound receptor complex composed of the BRASSINOSTEROID INSENSITIVE1 (BRI1) receptor kinase and BRI1-ASSOCIATED RECEPTOR KINASE1 (BAK1) [3] , [4] , [5] . Ligand-dependent auto- and trans -phosphorylation of BRI1 and BAK1 participate in receptor complex activation and modulate a cellular cascade of kinases and phosphatases [6] , [7] , which ultimately culminates in the dephosphorylation and activation of two transcription factors, BRASSINAZOLE-RESISTANT1 (BZR1) and BRI1-EMS SUPPRESSOR1 (BES1) [8] , [9] . BES1 and BZR1 bind to target promoters in the presence of different interacting partners to regulate BR genomic responses [10] , [11] , [12] . Adjustments in subcellular distribution of cell surface receptors are critical to modulate their signalling activity. Over the past decade, BRI1 has served as a model for a better understanding of the interplay between receptor trafficking, signal transduction and deactivation. BRI1 constitutively cycles between the plasma membrane and the trans -Golgi network/early endosome (TGN/EE), and it is targeted to the vacuole for degradation via the late endosomes/multivesicular bodies (MVB), independently of its ligand [13] , [14] . Internalization of BRI1 involves clathrin-mediated endocytosis, the adaptor complex AP-2 and the guanine exchange factor for ADP-ribosylation factor GTPase (ARF-GEFs) GNOM and GNL1 (refs 15 , 16 ). The drug-mediated trapping of BRI1 in endosomes was shown to enhance BR responses, leading to a model whereby BRI1 signals preferentially from endosomal compartments [13] . However, blocking BRI1 internalization by genetic or pharmacological interferences with AP2 was shown to activate BR signalling, indicating that BRI1 signals from the plasma membrane [15] , [16] . The post-translational modification of proteins involving ubiquitin (Ub) is well known in yeast and mammals to target proteins to proteasome-mediated degradation, and this involves K48-linked polyubiquitin chains [17] . Ubiquitination also serves numerous proteasome-independent roles, including the endocytosis of membrane proteins [18] . Notably, K63-linked polyubiquitin chains are essential for endosomal sorting and lysosome/vacuolar delivery of cargos via recognition by the ESCRT complex [19] . Ubiquitination also controls early steps of plasma membrane protein internalization. In yeast, Ub-mediated internalization is the major mechanism allowing retrieval of plasma membrane proteins [20] , while several other redundant Ub-independent pathways exist in mammals [21] . In plants, Ub-mediated endocytosis emerged only very recently with the study of ion and hormone transporters [22] , [23] , [24] , [25] , [26] . To date, the role of ubiquitination in the dynamics of plant transporters appears restricted to their targeting to the vacuole [23] , [24] . Whether Ub-mediated endocytosis has also been co-opted for driving the trafficking of other types of plant plasma membrane proteins, such as receptors, and for triggering early steps of internalization from the cell surface is unclear. Although several plant E3 ubiquitin ligases have been shown to interact with receptors [27] , [28] , [29] , [30] , their direct role in receptor ubiquitination has not been shown. Only the ubiquitination of the cell-surface flagellin receptor FLS2 by the PUB12 and PUB13 E3 ligases has been experimentally demonstrated; however, its link with FLS2 endocytosis is still undocumented [31] . Here we demonstrate that BRI1 is post-translationally modified by K63 polyubiquitin chains in vivo . Artificial ubiquitination of BRI1 negatively regulates its activity by enhanced vacuolar targeting from TGN/EE. Mass spectrometry analyses identify residue K866 of BRI1 as a target of ubiquitination in vivo . Loss of BRI1 ubiquitination at residue K866 is associated with subtle BR hypersensitivity, confirming the negative role of BRI1 ubiquitination on BR signalling, and pointing to the existence of other ubiquitination sites in BRI1. Model-based prediction of cell surface-exposed lysine residues in BRI1 allowed the generation of a functional but ubiquitination-defective BRI1. Global loss of BRI1 ubiquitination is associated with major defects in endosomal sorting and vacuolar delivery. In addition, using total internal reflection fluorescence microscopy (TIRF), we also shed light on the role of BRI1 ubiquitination in the BRI1 internalization from the cell surface. Altogether, our results identify K63-linked polyubiquitin chain formation as a dual targeting signal for BRI1 internalization and sorting along the endocytic pathway, and uncover its role in hormonally controlled plant development. BRI1 receptor is ubiquitinated in vivo Earlier work demonstrated that BRI1 undergoes endocytosis and trafficking to the vacuole, independently of its activation state [13] . However, little is known about the mechanisms driving BRI1 protein dynamics in the cell. Ubiquitination of cell-surface receptors in yeast and mammals has been shown to control internalization and/or vacuolar/lysosomal targeting [18] . To investigate BRI1 ubiquitination and its possible role in BR signalling, we used previously characterized transgenic lines expressing the functional BRI1–mCitrine fusion protein in complemented bri1 null mutants [32] , or in its isogenic wild-type background [33] , under the control of BRI1 promoter to reach endogenous expression level ( Supplementary Fig. 1a ). We first used anti-GFP antibodies to immunoprecipitate BRI1 from BRI1–mCitrine-expressing plants or wild-type plants as control. Immunoprecipitates from BRI1–mCitrine-expressing plants were enriched in BRI1–mCitrine, as attested by the strong signal observed at the expected size of BRI1–mCitrine fusion protein (~170 kDa; Fig. 1 , top left panel). To evaluate whether a fraction of BRI1 is post-translationally modified by ubiquitination, immunoprecipitates were probed with the general P4D1 anti-ubiquitin antibodies that recognize monoubiquitin and several forms of polyubiquitin chains. A high molecular weight smear, typical of ubiquitinated proteins, was specifically observed from ~170 kDa and higher in immunoprecipitates from BRI1–mCitrine plants ( Fig. 1 , top right panel). A comparable high molecular weight smear was observed when using the widely used Apu3 K63 polyubiquitin chain-specific antibody [34] , indicating that BRI1 is decorated by K63 polyubiquitin chains in vivo ( Fig. 1 , bottom left panel). In contrast, BRI1 immunoprecipitates showed no signal when probed with a K48 polyubiquitin chain-specific Apu2 antibody [34] , highlighting the fact that BRI1 does not carry K48-linked polyubiquitin chains ( Fig. 1 , bottom right panel). 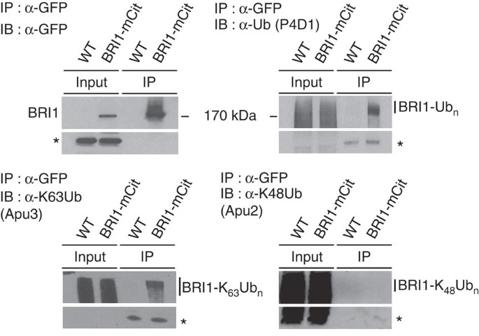Figure 1: BRI1 carries K63 polyubiquitin chainsin vivo. In vivoubiquitination analyses of BRI1. Immunoprecipitation was performed using anti-GFP antibodies on solubilized protein extracts from wild-type and mono-insertional homozygous BRI1–mCitrine plants and subjected to immunoblotting with anti-GFP (top left), anti-Ub P4D1 (top right), anti-K63 polyUb Apu3 (bottom left) and anti-K48 polyUb Apu2 antibodies (bottom right). IB, immunoblotting; IP, immunoprecipitation. The asterisk indicates nonspecific signals used as loading control. Figure 1: BRI1 carries K63 polyubiquitin chains in vivo . In vivo ubiquitination analyses of BRI1. Immunoprecipitation was performed using anti-GFP antibodies on solubilized protein extracts from wild-type and mono-insertional homozygous BRI1–mCitrine plants and subjected to immunoblotting with anti-GFP (top left), anti-Ub P4D1 (top right), anti-K63 polyUb Apu3 (bottom left) and anti-K48 polyUb Apu2 antibodies (bottom right). IB, immunoblotting; IP, immunoprecipitation. The asterisk indicates nonspecific signals used as loading control. Full size image We next addressed whether ubiquitination of BRI1 was regulated by steroid hormone perception. Challenging BRI1–mCitrine-expressing plants for 1 h with 1 μM brassinolide (BL), the most active BR form, had no detectable effect on the ubiquitination profile of BRI1–mCitrine ( Fig. 2a ; Supplementary Fig. 1b ). This concentration and duration of treatment is routinely used to monitor BR responses, such as the dephosphorylation of BES1 and BZR1 transcription factors [11] , [35] , [36] , [37] , suggesting that BRI1 ubiquitination does not correlate with ligand binding. It is possible however that under our growth conditions such young growing BRI1–mCitrine plants have close-to-maximal levels of activated receptors, thus preventing the detection of ligand-dependent changes in BRI1 ubiquitination. Two lines of evidence argue against this hypothesis. First, BRI1–mCitrine plants are fully responsive to exogenously applied BL, as observed by the marked change in BES1 phosphorylation status ( Supplementary Fig. 1c ), indicating that BR responses are not saturated. Second, growing plants on the BR biosynthetic inhibitor brassinazole (BRZ) to deplete the endogenous pool of BRs before a 1-h-BL treatment had no effect on BRI1 ubiquitination ( Supplementary Fig. 1d,e ). Interestingly, a 15-min-BL treatment revealed a modest increase in BRI1 ubiquitination ( Supplementary Fig. 1f,g ). Such a short BL treatment was sufficient to trigger total dephosphorylation of BES1 ( Supplementary Fig. 1h ), highlighting the fact that BRI1 kinase is activated within minutes after ligand binding. Altogether, these observations indicate that BRI1 ubiquitination appears to be largely independent of ligand binding with its regulation by BRs restricted to early BR receptor complex activation. 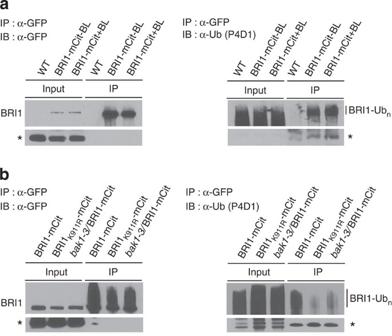Figure 2: BRI1 is ubiquitinated largely independently of ligand binding. (a) Ligand dependency of BRI1 ubiquitination. Ubiquitination assays were performed on wild-type and BRI1–mCitrine plants treated with mock (−BL) or 1 μM BL (+BL) for 1 h. The asterisk indicates nonspecific signals used as loading control. (b) BRI1 ubiquitination in mutants affected in receptor complex activation. Ubiquitination assays were performed on mono-insertional homozygous BRI1–mCitrine, kinase-dead BRI1K911R–mCitrine andbak1-3/BRI1–mCitrine lines. The asterisk indicates nonspecific signals used as loading control. Figure 2: BRI1 is ubiquitinated largely independently of ligand binding. ( a ) Ligand dependency of BRI1 ubiquitination. Ubiquitination assays were performed on wild-type and BRI1–mCitrine plants treated with mock (−BL) or 1 μM BL (+BL) for 1 h. The asterisk indicates nonspecific signals used as loading control. ( b ) BRI1 ubiquitination in mutants affected in receptor complex activation. Ubiquitination assays were performed on mono-insertional homozygous BRI1–mCitrine, kinase-dead BRI1 K911R –mCitrine and bak1-3 /BRI1–mCitrine lines. The asterisk indicates nonspecific signals used as loading control. Full size image Mechanism of BRI1 ubiquitination We next investigated the molecular mechanisms driving BRI1 ubiquitination. In particular, we focused on the possible role played by receptor activation, although BRI1 ubiquitination appears to be mostly independent of ligand binding. Lysine residue K911 of BRI1 is an invariant residue in subdomain II of kinases and is critical for BRI1 kinase activity and BR signalling. Consequently, bri1 mutant expressing the kinase-dead K911R mutation is not complemented and show extreme dwarfism [38] . Transgenic plants expressing the non-functional BRI1 K911R mutant form under the control of the BRI1 promoter were assayed for BRI1 ubiquitination. Care was taken to normalize the immunoprecipitation carried out from BRI1–mCitrine- and BRI1 K911R –mCitrine-expressing plants to compensate for difference in transgene expression level. In contrast to what is observed for the wild-type form of BRI1, BRI1 K911R -expressing plants showed reduced ubiquitination ( Fig. 2b , Supplementary Fig. 1i ). This suggests that BRI1 kinase activity is required for BRI1 ubiquitination. The possibility that residue K911 itself is a major ubiquitination site in the BRI1 protein is very unlikely, since it is not surface-exposed ( Supplementary Fig. 5a ). Mutation in K911 of BRI1 was shown to drastically affect BRI1–BAK1 receptor complex formation [39] . We therefore addressed whether the co-receptor BAK1 was also required for BRI1 ubiquitination. To this purpose, we expressed BRI1–mCitrine in a bak1 null mutant background. bak1-3 /BRI1–mCitrine showed a reduction in BRI1 ubiquitination compared with BRI1–mCitrine plants, although not statistically significant ( Fig. 2b , Supplementary Fig. 1i ). The defect in BRI1 ubiquitination observed in bak1-3 is less severe than what is observed for kinase-dead BRI1, likely because of genetic redundancy with other BAK1 homologues [40] . The defect of BRI1 ubiquitination observed in genetic backgrounds impaired in receptor complex activation is however not explained by a different subcellular distribution of BRI1 in the cell. BRI1 is indeed found both at the plasma membrane and in endosomal compartments in BRI1–mCitrine and bak1-3 /BRI1–mCitrine, as well as in BRI1 K911R –mCitrine plants, although the expression level of kinase-dead BRI1 is very low ( Supplementary Fig. 1j ). Altogether, these results indicate that, although BRI1 ubiquitination is largely independent of steroid binding, it requires BRI1 kinase activity and, to a lesser extent, its co-receptor BAK1—two hallmarks of ligand perception by BRI1 (ref. 1 ). BRI1 artificial ubiquitination triggers vacuolar targeting Extensive work in yeast and mammals demonstrated the importance of mono- and K63 polyubiquitination for plasma membrane protein internalization, and sorting in MVB [20] , [41] . However, K63 polyubiquitination has also been involved in the regulation of kinases. TAK1 (transforming growth factor-β activating kinase 1) mediates NF-κB activation in response to the activation of the TGF-β receptor. Upon stimulation with TGF-β, TAK1 undergoes TRAF6-dependent K63-linked ubiquitination on residue K34. Modification of TAK1 by ubiquitination is critical for TAK1 autophosphorylation and subsequent activation [42] . To get a first glimpse into the biological role of BRI1 post-translational modification by K63 polyubiquitination, we took a gain-of-function approach where BRI1–mCitrine was translationally fused to a single Ub moiety. Although BRI1 is artificially linked to a single Ub, seven lysine residues are found in Ub including lysine K63 that may engage in K63 polyUb chain formation. We used the complementation of the dwarfism of the bri1 null T-DNA knockout mutant [32] , as readout for BRI1 activity ( Supplementary Fig. 2a ). As controls, we also generated bri1 /BRI1–mCitrine, as well as bri1 /BRI1–mCitrine–Ub I44A carrying a point mutation in a hydrophobic patch necessary for recognition by ubiquitin-binding domain proteins [43] . Care was taken at that stage to use transgenic lines expressing similar amounts of RNA for the respective transgenes ( Supplementary Fig. 2b ). Both bri1 /BRI1–mCitrine and bri1 /BRI1–mCitrine–Ub I44A, expressing a non-functional ubiquitin, fully complemented the severe dwarfism of bri1 null mutant ( Fig. 3a ). In contrast, BRI1–mCitrine–Ub did not complement the bri1 phenotype, indicating that artificial ubiquitination of BRI1 downregulates its activity. Artificial ubiquitination of BRI1–mCitrine protein led to a strong decrease in total BRI1 protein levels compared with wild-type BRI1–mCitrine and BRI1–mCitrine–Ub I44A ( Fig. 3b , Supplementary Fig. 2c ). Confocal microscopy observations, using similar detection settings to compare the fluorescence levels of the three transgenic lines and to quantify total fluorescence intensity, clearly indicate that BRI1–mCitrine–Ub fails to accumulate in the cell ( Fig. 3c,d ). Higher laser intensity and gain, however, allowed the detection of close-to-background levels of BRI1–mCitrine–Ub as punctate pattern, with little or no accumulation at the plasma membrane ( Fig. 3c , inset). 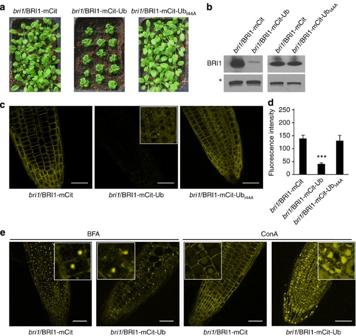Figure 3: Artificial ubiquitination of BRI1 triggers vacuolar targeting from TGN/EE. (a) Phenotypic analysis of transgenic plants expressing BRI1–mCitrine, BRI1–mCitrine–Ub and BRI1–mCitrine–UbI44Ain thebri1null background. All transgenic lines are mono-insertional and homozygous for the transgene. A representative transgenic line is shown for each genotype. (b) Western blot analyses monitoring BRI1 protein accumulation inbri1/BRI1–mCitrine,bri1/BRI1–mCitrine–Ub andbri1/BRI1–mCitrine–UbI44Aplants using anti-GFP antibodies. The asterisk indicates nonspecific signals used as loading control. (c) Confocal microscopy analyses ofbri1/BRI1–mCitrine,bri1/BRI1–mCitrine–Ub andbri1/BRI1–mCitrine–UbI44Aroots. Similar confocal detection settings were used to compare the different lines. Inset, higher laser power and gain to visualize BRI1–mCitrine–Ub. Scale bars=50 μm. (d) Quantification of the total fluorescence intensity ofbri1/BRI1–mCitrine,bri1/BRI1–mCitrine–Ub andbri1/BRI1–mCitrine–UbI44Aroots. Experiments were conducted in triplicates. Error bars represent s.d. (n=15). The asterisks indicate a statistically significant difference betweenbri1/BRI1–mCit–Ub and thebri1/BRI1–mCit control by Kruskal–Wallis one-way analysis of variance and Dunnett multiple testing (P<0.0001). (e) Drug sensitivity ofbri1/BRI1–mCitrine andbri1/BRI1–mCitrine–Ub plants. Plants were exposed to BFA (50 μM) and ConA (2 μM) for 1 h. Similar confocal detection settings were used to compare the different lines. Inset, higher magnification to visualize the accumulation of BRI1–mCitrine and BRI1–mCitrine–Ub fluorescent proteins in BFA bodies and vacuoles upon BFA and ConA treatment, respectively. Scale bars=50 μm. Figure 3: Artificial ubiquitination of BRI1 triggers vacuolar targeting from TGN/EE. ( a ) Phenotypic analysis of transgenic plants expressing BRI1–mCitrine, BRI1–mCitrine–Ub and BRI1–mCitrine–Ub I44A in the bri1 null background. All transgenic lines are mono-insertional and homozygous for the transgene. A representative transgenic line is shown for each genotype. ( b ) Western blot analyses monitoring BRI1 protein accumulation in bri1 /BRI1–mCitrine, bri1 /BRI1–mCitrine–Ub and bri1 /BRI1–mCitrine–Ub I44A plants using anti-GFP antibodies. The asterisk indicates nonspecific signals used as loading control. ( c ) Confocal microscopy analyses of bri1 /BRI1–mCitrine, bri1 /BRI1–mCitrine–Ub and bri1 /BRI1–mCitrine–Ub I44A roots. Similar confocal detection settings were used to compare the different lines. Inset, higher laser power and gain to visualize BRI1–mCitrine–Ub. Scale bars=50 μm. ( d ) Quantification of the total fluorescence intensity of bri1 /BRI1–mCitrine, bri1 /BRI1–mCitrine–Ub and bri1 /BRI1–mCitrine–Ub I44A roots. Experiments were conducted in triplicates. Error bars represent s.d. ( n =15). The asterisks indicate a statistically significant difference between bri1 /BRI1–mCit–Ub and the bri1 /BRI1–mCit control by Kruskal–Wallis one-way analysis of variance and Dunnett multiple testing ( P <0.0001). ( e ) Drug sensitivity of bri1 /BRI1–mCitrine and bri1 /BRI1–mCitrine–Ub plants. Plants were exposed to BFA (50 μM) and ConA (2 μM) for 1 h. Similar confocal detection settings were used to compare the different lines. Inset, higher magnification to visualize the accumulation of BRI1–mCitrine and BRI1–mCitrine–Ub fluorescent proteins in BFA bodies and vacuoles upon BFA and ConA treatment, respectively. Scale bars=50 μm. Full size image To investigate deeper the mechanisms driving the loss of BRI1–mCitrine–Ub protein, we took advantage of drugs interfering with vesicular trafficking. The fungal toxin Brefeldin A (BFA) is a widely used inhibitor of endosomal trafficking, creating large aggregates of trans -Golgi network/early endosomal compartments in the Arabidopsis root. Although BRI1–mCitrine–Ub failed to accumulate under normal conditions, BRI1–mCitrine–Ub levels rapidly built up in BFA bodies after BFA treatment to reach the levels observed for BRI1–mCitrine ( Fig. 3e , Supplementary Fig. 3a ). This suggests that BRI1–mCitrine–Ub is translated, exits the endoplasmic reticulum and passes through the TGN/EE on its way to degradation. We next assessed the influence of the vacuolar ATPase inhibitor Concanamycin A (ConA), which prevents the degradation of proteins targeted to the vacuole [44] . ConA treatment led to the dramatic accumulation of BRI1–mCitrine–Ub in the vacuole ( Fig. 3e , Supplementary Fig. 3b ), compared with BRI1–mCitrine, thus revealing enhanced vacuolar delivery triggered by ubiquitin. This indicates that artificial ubiquitination of BRI1–mCitrine is sufficient for vacuolar targeting, consistent with what has been recently observed for other plant cargos [24] , [45] , [46] . We next investigated whether BRI1–mCitrine–Ub was trafficking via the plasma membrane on its way to the vacuole by inhibiting clathrin-mediated endocytosis, the major endocytic road in plants [47] . Treatment with the inhibitor of clathrin-mediated endocytosis, TyrA23, was ineffective at stabilizing BRI1–mCitrine–Ub at the cell surface, but rather led to a cytosolic-like pattern of fluorescence ( Supplementary Fig. 3c ). In contrast, TyrA23 prevented the formation of BFA bodies in BRI1–mCitrine plants ( Supplementary Fig. 3d ), attesting that TyrA23 treatment was active. Taken together, these results indicate that artificial ubiquitination is recognized before reaching the plasma membrane, likely at the TGN/EE, and serves as a targeting signal for degradation in the vacuole. To discriminate further the form of Ub associated with vacuolar targeting, we generated bri1 /BRI1–mCitrine–Ub 7KR plants where all seven lysines from Ub were mutated to arginines to prevent K63 polyubiquitin chain formation. Confocal microscopy observations of bri1 /BRI1–mCitrine and bri1 /BRI1–mCitrine–Ub 7KR using the same detection settings showed that artificial monoubiquitination of BRI1 also impairs BRI1 protein accumulation ( Supplementary Fig. 3e,f ). Monoubiquitination of BRI1 therefore appears sufficient to trigger its vacuolar delivery, similarly to what has been reported for the plant ATPase phorbol myristate acetate or the yeast polyphosphate endophosphatase Phm5 (refs 45 , 48 ). BRI1 is ubiquitinated at residue K866 in vivo To identify ubiquitination sites in BRI1, we performed immunoprecipitation of BRI1 in the presence of deubiquitinase inhibitors followed by mass spectrometry analyses. Immunopurified BRI1–mCitrine was digested by trypsin and subjected to liquid chromatography tandem mass spectrometry analyses (LC-MS/MS). Multidimensional protein identification technology analyses on BRI1–mCitrine immunoprecipitates detected nine BRI1 peptides, including the EALSINLAAFEK GG PLR peptide modified by the tryptic ubiquitin remnant G–G isopeptide on the lysine residue K866. This residue lies on the cytosolic face of the BRI1 protein, in the juxtamembrane domain ( Fig. 4a ). To examine the biological role of K866 ubiquitination, we generated transgenic plants expressing BRI1 where residue K866 is substituted by the positively charged but nonubiquitinatable R residue (BRI1 K866R ), under the control of its own promoter in bri1 background. bri1 /BRI1 K866R –mCitrine transgenic plants expressing similar BRI1–mCitrine levels than bri1 /BRI1–mCitrine showed no macroscopic phenotypes at the adult stage ( Fig. 4b,c ). To better characterize BRI1 K866R -expressing plants, we monitored two well-established readouts of BR signalling such as the phosphorylation state of BES1 and hypocotyl length. Compared with plants expressing wild-type BRI1, BRI1 K866R -expressing plants reproducibly showed more dephosphorylated BES1 ( Fig. 4c ; Supplementary Fig. 4a ) and longer hypocotyls when grown under both normal conditions and BRZ ( Fig. 4d ). These observations suggest that expression of BRI1 K866R leads to a mild activation of BR signalling. No striking difference on the localization and the levels of the BRI1 K866R –mCitrine protein could be observed ( Fig. 4e ). Altogether, ubiquitination of residue K866 appears to play a negative role on BRI1 activity. The fact that bri1 /BRI1 K866R –mCitrine transgenic plants only show a slight activation of BR signalling compared with what has been reported for BRI1-overexpressing plants [33] , and still harbours massive ubiquitination ( Supplementary Fig. 4b,c ) suggests that many more ubiquitination sites exist in BRI1. 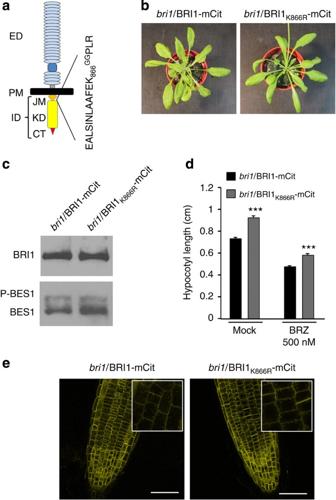Figure 4: Ubiquitination of residue K866 negatively regulates BRI1. (a) Identification ofin vivoubiquitination sites in BRI1. ED, extracellular domain; PM, plasma membrane, ID, intracellular domain; JM, juxtamembrane domain; KD, kinase domain; CT, C-terminal domain. The ubiquitinated peptide carrying the GG di-glycine signature on K866 is shown. (b) Phenotypic analysis of 4-week-old mono-insertional homozygousbri1/BRI1-mCitrine andbri1/BRI1K866R-mCitrine plants. A representative transgenic line is shown for both genotypes (c) Western blot analyses onbri1/BRI1-mCitrine andbri1/BRI1K866R-mCitrine plants. Protein levels were detected with anti-GFP and anti-BES1 antibodies, respectively. (d) Average hypocotyl lengths of 3-day-old etiolatedbri1/BRI1-mCitrine andbri1/BRI1K866R-mCitrine seedlings. Experiments were done in triplicates. Error bars indicate standard deviation (n=15). The asterisks indicate a statistically significant difference betweenbri1/BRI1-mCit and thebri1/BRI1K866R-mCit control (Mann-Whitney,P<0.0001). (e) Confocal microscopy analyses ofbri1/BRI1-mCitrine andbri1/BRI1K866R-mCitrine roots. Similar confocal detection settings were used to compare the two representative transgenic lines. Inset, higher magnification. Scale bars=50 μm. Figure 4: Ubiquitination of residue K866 negatively regulates BRI1. ( a ) Identification of in vivo ubiquitination sites in BRI1. ED, extracellular domain; PM, plasma membrane, ID, intracellular domain; JM, juxtamembrane domain; KD, kinase domain; CT, C-terminal domain. The ubiquitinated peptide carrying the GG di-glycine signature on K866 is shown. ( b ) Phenotypic analysis of 4-week-old mono-insertional homozygous bri1 /BRI1-mCitrine and bri1 /BRI1 K866R -mCitrine plants. A representative transgenic line is shown for both genotypes ( c ) Western blot analyses on bri1 /BRI1-mCitrine and bri1 /BRI1 K866R -mCitrine plants. Protein levels were detected with anti-GFP and anti-BES1 antibodies, respectively. ( d ) Average hypocotyl lengths of 3-day-old etiolated bri1 /BRI1-mCitrine and bri1 /BRI1 K866R -mCitrine seedlings. Experiments were done in triplicates. Error bars indicate standard deviation ( n =15). The asterisks indicate a statistically significant difference between bri1 /BRI1-mCit and the bri1 /BRI1 K866R -mCit control (Mann-Whitney, P <0.0001). ( e ) Confocal microscopy analyses of bri1 /BRI1-mCitrine and bri1 /BRI1 K866R -mCitrine roots. Similar confocal detection settings were used to compare the two representative transgenic lines. Inset, higher magnification. Scale bars=50 μm. Full size image Loss of BRI1 ubiquitination impairs endocytosis and sorting The intracellular domain of BRI1 contains 29 lysine residues. Sequence alignment of BRI1 with (i) the BRI1-like homologues from Arabidopsis , (ii) BRI1 from other plant species, (iii) Arabidopsis receptor kinases belonging to different subfamilies such as FLS2 and CLV1 and (iv) human IRAK4 indicates that four lysines from BRI1 kinase are highly conserved in all kinases analysed. These include the ATP-binding pocket-located K899, K911 and K912, and residue K1011 in the catalytic loop, which are mostly buried in the recently resolved BRI1 kinase structure [49] ( Supplementary Fig. 5a ), and are likely critical for kinase activity since highly conserved. To pinpoint the role of BRI1 ubiquitination, we sought to generate an ubiquitination-defective BRI1 that retains its kinase activity. We therefore mutated 25 lysines to arginines in BRI1 intracellular domain, and kept only the four strictly conserved lysine residues K899, K911, K912 and K1011. Expression of the resulting BRI1 25KR mutants under the control of BRI1 promoter complemented the dwarf phenotype of bri1 null mutant ( Fig. 5a ). This result indicates that BRI1 25KR –mCitrine was still functional and that none of these 25 lysines are required for receptor activation. BRI1 25KR –mCitrine-expressing plants were severely compromised for BRI1 ubiquitination compared with BRI1–mCitrine ( Supplementary Fig. 5b,c ). Interestingly, BRI1 25KR -expressing plants showed long bending petioles and narrow leaf blades ( Fig. 5a,b ; Supplementary Fig. 5d ), reminiscent of what is observed in BRI1 overexpressors [33] . This correlates with increased accumulation of dephosphorylated BES1, which positively regulates BR signalling [1] ( Fig. 5c,d ). The BR hypersensitivity phenotype of BRI1 25KR is observed for plants that express less BRI1 proteins than bri1 /BRI1–mCitrine plants ( Fig. 5c,d ), highlighting further the negative role played by ubiquitination on BRI1 activity. 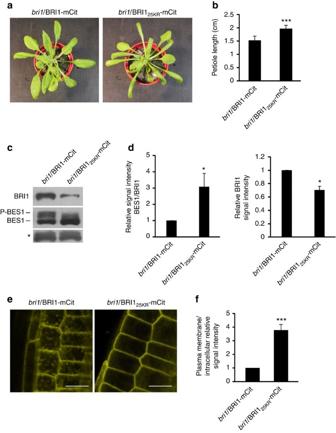Figure 5: BRI1 ubiquitination controls brassinosteroid signalling and BRI1 localization. (a) Phenotypic analysis of 4-week-oldbri1/BRI1–mCitrine andbri1/BRI125KR–mCitrine mono-insertional homozygous plants. A representative transgenic line is shown for both genotypes. (b) Average petiole lengths of the fourth true leaf from 4-week-oldbri1/BRI1–mCitrine andbri1/BRI125KR–mCitrine plants. Experiments were carried out in triplicates. Error bars represent s.d. (n=20). The asterisk indicates a statistically significant difference betweenbri1/BRI1–mCit and thebri1/BRI125KR–mCit control (Mann–Whitney,P<0.0001). (c) Western blot analyses onbri1/BRI1–mCitrine andbri1/BRI125KR–mCitrine plants using anti-GFP and anti-BES1 antibodies. The asterisk indicates nonspecific signals used as loading control. (d) Quantification of dephosphorylated BES1 (left) and BRI1 (right) protein levels inbri/BRI1–mCit andbri1/BRI125KR–mCit. Experiments were carried out in triplicates. Error bars represent s.d. (n=3). The asterisk indicates a statistically significant difference in dephosphorylated BES1 and BRI1 levels betweenbri1/BRI1–mCit andbri1/BRI125KR–mCit (Mann–Whitney,P<0.05). (e) Confocal microscopy analyses ofbri1/BRI1–mCitrine andbri1/BRI125KR–mCitrine roots. Scale bars=7 μm. (f) Quantification of the ratio between plasma membrane and intracellular fluorescence signal intensities of BRI1–mCitrine and BRI125KR–mCitrine. Experiments were carried out in triplicates. Error bars represent s.d. (n=15). The asterisk indicates a statistically significant difference betweenbri1/BRI1–mCit and thebri1/BRI125KR–mCit (Mann-Whitney,P<0.0005). Figure 5: BRI1 ubiquitination controls brassinosteroid signalling and BRI1 localization. ( a ) Phenotypic analysis of 4-week-old bri1 /BRI1–mCitrine and bri1 /BRI1 25KR –mCitrine mono-insertional homozygous plants. A representative transgenic line is shown for both genotypes. ( b ) Average petiole lengths of the fourth true leaf from 4-week-old bri1 /BRI1–mCitrine and bri1 /BRI1 25KR –mCitrine plants. Experiments were carried out in triplicates. Error bars represent s.d. ( n =20). The asterisk indicates a statistically significant difference between bri1 /BRI1–mCit and the bri1 /BRI1 25KR –mCit control (Mann–Whitney, P <0.0001). ( c ) Western blot analyses on bri1 /BRI1–mCitrine and bri1 /BRI1 25KR –mCitrine plants using anti-GFP and anti-BES1 antibodies. The asterisk indicates nonspecific signals used as loading control. ( d ) Quantification of dephosphorylated BES1 (left) and BRI1 (right) protein levels in bri /BRI1–mCit and bri1 /BRI1 25KR –mCit. Experiments were carried out in triplicates. Error bars represent s.d. ( n =3). The asterisk indicates a statistically significant difference in dephosphorylated BES1 and BRI1 levels between bri1 /BRI1–mCit and bri1 /BRI1 25KR –mCit (Mann–Whitney, P <0.05). ( e ) Confocal microscopy analyses of bri1 /BRI1–mCitrine and bri1 /BRI1 25KR –mCitrine roots. Scale bars=7 μm. ( f ) Quantification of the ratio between plasma membrane and intracellular fluorescence signal intensities of BRI1–mCitrine and BRI1 25KR –mCitrine. Experiments were carried out in triplicates. Error bars represent s.d. ( n =15). The asterisk indicates a statistically significant difference between bri1 /BRI1–mCit and the bri1 /BRI1 25KR –mCit (Mann-Whitney, P <0.0005). Full size image The BRI1 protein is found under normal conditions at the plasma membrane, but also in endosomal compartments (TGN/EE and MVB; Fig. 5e ) [13] , [14] . In contrast, BRI1 25KR –mCitrine was found mostly at the cell surface, with little intracellular compartments observed ( Fig. 5e,f ). To unravel the mechanism leading the different intracellular distribution of BRI1 25KR –mCitrine, we compared the endocytic trafficking of BRI1–mCitrine and BRI1 25KR –mCitrine. BFA inhibits the trafficking of membrane proteins from TGN/EE to MVB and recycling to the plasma membrane, but allows endocytosis. Both BRI1–mCitrine and BRI1 25KR –mCitrine accumulated in BFA compartments in absence of de novo protein synthesis ( Fig. 6a,b ), although the size of BFA bodies appeared smaller for BRI1 25KR –mCitrine ( Fig. 6c ). This suggests that BRI1 25KR –mCitrine undergoes internalization from the plasma membrane, but presumably to a lesser extent than its wild-type counterpart so that less BRI1 protein is trapped in BFA bodies. To obtain more resolution and quantitative data on the dynamics of BRI1 and BRI1 25KR at the cell surface, we implemented TIRF. TIRF generates high-contrast images and allows studying the dynamic behaviour of proteins at the plasma membrane. We were unable to perform reproducible TIRF imaging at the root tip likely because of the ovoid shape of the root tip and the presence of root hairs in root samples, preventing good contacting with the coverslip, a prerequisite for TIRF imaging. Hypocotyls from etiolated seedlings have flat cells suited with TIRF imaging and their elongation strongly depends on BR perception by BRI1 (ref. 1 ). BRI1–mCitrine localized to the plasma membrane in etiolated hypocotyl cells, but the TGN/EE pool of BRI1 was difficult to observe because of the large central vacuole ( Supplementary Fig. 6a ). BRI1 trafficking was found to be sensitive to BFA in etiolated hypocotyl cells, as highlighted by the intracellular aggregation of BRI1–mCitrine upon BFA treatment. Finally, artificially ubiquitinated BRI1 failed to accumulate in hypocotyl cells. Altogether, this indicates that BRI1 trafficking in etiolated hypocotyl cells mirrors what has been described in roots. BRI1–mCitrine-expressing plants were therefore imaged using TIRF microscopy over time and showed small diffraction-limited fluorescent spots ( Supplementary Movies 1,2 ). These spots were immobile on the ( x , y ) axis but dynamically appeared and disappeared from the focal plane, thus representing fusion and fission events at the cell surface. A similar pattern was observed for BRI1 25KR –mCitrine, although the density of spots at the cell surface was higher ( Supplementary Fig. 6b ). To grasp the role of ubiquitination in BRI1 internalization from the plasma membrane, we further analysed the dynamic behaviour of wild-type BRI1 and BRI1 25KR using kymograph analysis. Kymographs monitor on a single image the intensity at a given ( x , y ) location over time, and allow determination of surface time residence for wild-type BRI1 and BRI1 25KR by measuring track length ( Fig. 6d ). The time of residency of BRI1–mCitrine at the cell surface was widely distributed ( Fig. 6e ), but over 60% of the spots resided less than 10 s at the plasma membrane. The distribution observed for BRI1 25KR was markedly different, with most spots persisting longer at the plasma membrane. The surface residence time median values for BRI1 and BRI1 25KR were 7.2 and 28.6 s, respectively ( Supplementary Fig. 6c ). These observations clearly argue for a direct role of BRI1 ubiquitination in internalization from the plasma membrane. 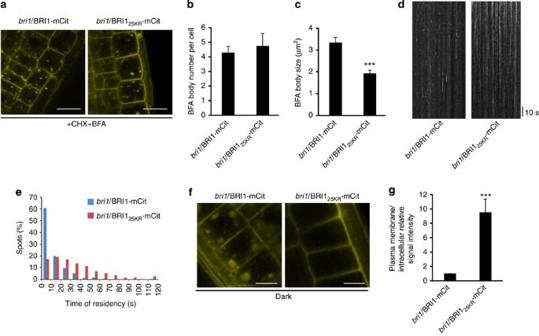Figure 6: Loss of BRI1 ubiquitination impairs its internalization and vacuolar targeting. (a) Sensitivity ofbri1/BRI1–mCitrine andbri1/BRI125KR–mCitrine plants to BFA. Plants were pretreated with 100 μM CHX for 1 h and exposed to 100 μM CHX and 50 μM BFA for 1 h. Scale bars=7 μm. (b) Quantification of BFA body number inbri1/BRI1–mCit andbri1/BRI125KR–mCit roots. Experiments were carried out in triplicates. Error bars represent s.d. (n=15). No statistical difference if observed betweenbri1/BRI1–mCit andbri1/BRI125KR–mCit (Mann–Whitney,P>0.05). (c) Quantification of BFA body size inbri1/BRI1–mCit andbri1/BRI125KR–mCit roots. Experiments were carried out in triplicates. Error bars represent s.d. (n=15). The asterisk indicates a statistically significant difference between the two genotypes (Mann–Whitney,P<0.0001). (d) Kymograph analysis from TIRF movies ofbri1/BRI1–mCitrine andbri1/BRI125KR–mCitrine. The timescale is shown. (e) Time of residency at the plasma membrane ofbri1/BRI1–mCitrine andbri1/BRI125KR–mCitrine. The distribution was obtained from kymograph-based track length analyses (n=350). (f) Sensitivity of BRI1–mCitrine and BRI125KR–mCitrine to dark growth conditions. Light-grown seedlings were kept in the dark for 2 h before confocal imaging. Scale bars=7 μm. (g) Quantification of the ratio between relative plasma membrane and intracellular fluorescence signal intensities of BRI1–mCitrine and BRI125KR–mCitrine. Experiments were carried out in triplicates. Error bars represent s.d. (n=15). The asterisk indicates a statistically significant difference between BRI1–mCit and the BRI125KR–mCit (Mann–Whitney,P<0.0001). Figure 6: Loss of BRI1 ubiquitination impairs its internalization and vacuolar targeting. ( a ) Sensitivity of bri1 /BRI1–mCitrine and bri1 /BRI1 25KR –mCitrine plants to BFA. Plants were pretreated with 100 μM CHX for 1 h and exposed to 100 μM CHX and 50 μM BFA for 1 h. Scale bars=7 μm. ( b ) Quantification of BFA body number in bri1 /BRI1–mCit and bri1 /BRI1 25KR –mCit roots. Experiments were carried out in triplicates. Error bars represent s.d. ( n =15). No statistical difference if observed between bri1 /BRI1–mCit and bri1 /BRI1 25KR –mCit (Mann–Whitney, P >0.05). ( c ) Quantification of BFA body size in bri1 /BRI1–mCit and bri1 /BRI1 25KR –mCit roots. Experiments were carried out in triplicates. Error bars represent s.d. ( n =15). The asterisk indicates a statistically significant difference between the two genotypes (Mann–Whitney, P <0.0001). ( d ) Kymograph analysis from TIRF movies of bri1 /BRI1–mCitrine and bri1 /BRI1 25KR –mCitrine. The timescale is shown. ( e ) Time of residency at the plasma membrane of bri1 /BRI1–mCitrine and bri1 /BRI1 25KR –mCitrine. The distribution was obtained from kymograph-based track length analyses ( n =350). ( f ) Sensitivity of BRI1–mCitrine and BRI1 25KR –mCitrine to dark growth conditions. Light-grown seedlings were kept in the dark for 2 h before confocal imaging. Scale bars=7 μm. ( g ) Quantification of the ratio between relative plasma membrane and intracellular fluorescence signal intensities of BRI1–mCitrine and BRI1 25KR –mCitrine. Experiments were carried out in triplicates. Error bars represent s.d. ( n =15). The asterisk indicates a statistically significant difference between BRI1–mCit and the BRI1 25KR –mCit (Mann–Whitney, P <0.0001). Full size image We next monitored the role of ubiquitination in BRI1 vacuolar targeting. BRI1–mCitrine and BRI1 25KR –mCitrine were transferred to dark conditions, which impair vacuolar lytic activity and allow visualization of the pH-resistant mCitrine fluorescent fusion proteins targeted to the vacuole [50] , and monitored by confocal microscopy. Consistently, BRI1–mCitrine showed vacuolar accumulation after 2 h of darkness ( Fig. 6f,g ). However, BRI1 25KR –mCitrine exhibited no vacuolar targeting within the same time frame. Consistently, the ubiquitination-defective BRI1 25KR is more stable than wild-type BRI1 ( Supplementary Fig. 6d,e ). The inability of BRI1 25KR to reach the vacuole combined to the increased cell surface accumulation suggest that BRI1 25KR undergoes enhanced recycling to the cell surface. Endocytosed BRI1 protein was previously shown to recycle to the cell surface by BFA washout experiments [51] , in which the recovery of BRI1 at the plasma membrane is monitored after BFA removal in the absence of protein synthesis. We confirmed that BRI1 both recycles at the plasma membrane and is also targeted to the vacuole after BFA washout, and observed that BRI1 25KR recycles more to the cell surface ( Supplementary Fig. 6f,g ). Altogether, our results unravel the dual role of BRI1 ubiquitination in BRI1 receptor internalization from the plasma membrane and also in its endosomal sorting and vacuolar targeting. The BR receptor BRI1 is the best-studied plant receptor and serves as the archetypical receptor to study the activation/deactivation mechanisms involved in receptor-mediated signalling. Previous studies have shed light on the ligand-dependent oligomerization and phosphorylation of the BRI1/BAK1 receptor complex and have identified components of the BR signalling pathway controlling BR genomic responses [52] . However, not much is known about the mechanisms driving the trafficking of BRI1 and its turnover in relationship with signalling. In this report, we show that BRI1 dynamics in the cell is controlled by ubiquitination and unravel its role for BR-mediated plant growth. Ubiquitination of proteins has been associated with many different cellular outputs in yeast and mammals, depending on the type of ubiquitination [41] . In the case of membrane proteins, ubiquitination triggers endocytosis and vacuolar/lysosomal degradation [18] . In plants, only a handful of integral membrane proteins have been shown to undergo Ub-mediated endocytosis. These examples are so far exclusively restricted to multispan transporters involved in iron, boron or phosphate nutrition or in auxin transport [22] , [23] , [24] , [25] . Both monoubiquitination and K63 polyubiquitination have been implicated in these examples, consistent with their described roles in yeast and mammals. Ubiquitination of plant receptors is still poorly documented, although several E3-Ub ligases interacting with receptors have been identified [27] , [28] , [29] , [30] . Only the Flagellin receptor FLS2 involved in plant immune responses has been shown to be ubiquitinated [31] . However, FLS2 carries K48 polyubiquitin chains and has been suggested to be degraded by the proteasome. In this study, we first demonstrated using a gain-of-function approach that the artificial ubiquitination of BRI1 is sufficient for destabilizing the corresponding protein. Artificial monoubiquitination of BRI1 appeared sufficient to prevent accumulation of BRI1. Destabilization of the BRI1–mCitrine–Ub protein involves trafficking through the TGN/EE and degradation in the vacuole, based on the strong accumulation of BRI1–mCitrine–Ub following treatments with BFA and ConA. Inhibition of clathrin-mediated endocytosis, the major BRI1 endocytic route [15] , [16] , with TyrA23 failed to stabilize BRI1–mCitrine–Ub at the cell surface, suggesting that the artificially ubiquitinated BRI1 variant never reaches the plasma membrane. Formally, artificially ubiquitinated BRI1 could be rapidly endocytosed from the plasma membrane using a clathrin-independent TyrA23-insensitive pathway. However, we favour the hypothesis that BRI1–mCitrine–Ub is recognized at the TGN/EE and diverted away from the secretory pathway before it reaches the cell surface, being directly routed to the vacuole for degradation. In yeast and mammals, GGA proteins at the TGN work to divert ubiquitinated cargos from the secretory pathway towards endosomes, preventing them from reaching the cell surface [53] . Late endocytic sorting of ubiquitinated cargos in intraluminal vesicles of MVB and vacuolar/lysosomal targeting require the late endosome-located ESCRT complex [18] . In plants, the TOL GGA-related proteins and several subunits of the ESCRT complex have been recently detected in TGN/EE [54] , [55] , indicating that the sorting of artificially ubiquitinated BRI1 indeed occurs at the TGN/EE. We demonstrated that BRI1 is K63 polyubiquitinated in vivo , and does not carry K48 polyubiquitin chains. The combination of ubiquitination site identification by mass spectrometry and model-based prediction allowed us to generate a functional ubiquitination-defective BRI1 25KR mutant form. In contrast to wild-type BRI1 that shows significant endosomal localization [13] , BRI1 25KR was mostly found at the cell surface. To decipher whether the increased plasma membrane localization resulted from internalization defects and/or intracellular sorting defects, we implemented TIRF microscopy to specifically monitor BRI1 dynamics at the cell surface. Such analysis first highlighted the highly dynamic behaviour of wild-type BRI1, with extremely rapid fusion and fission events within the seconds range. Interestingly, BRI1 25KR shows much slower fusion/fission events at the plasma membrane, within the tens of second range, indicating that ubiquitination of BRI1 triggers its internalization from the cell surface. Detailed analysis of BRI1 25KR trafficking also highlighted the crucial role of ubiquitination in BRI1 intracellular sorting and vacuolar targeting. Overall, ubiquitination of BRI1 therefore appears as one several redundant mechanisms driving BRI1 internalizing from the plasma membrane, whereas it is absolutely essential for BRI1 endosomal sorting ( Fig. 7 ). The combination of both slower internalization and forced recycling caused by vacuolar targeting defects are therefore the basis of increased BRI1 25KR at the cell surface and increased spot density. This scenario is reminiscent of what is currently debated for the epidermal growth factor receptor (EGFR) in animals. Mutation of 15 ubiquitin conjugation sites found in the EGFR kinase domain or the Cbl E3 ligase-binding site does not affect EGFR internalization, although preventing lysosomal degradation [56] . EGFR internalization from the cell surface is impaired only when 21 lysine residues in the kinase domain and C-terminal domain are mutated, although the three distal lysines in the C-terminal domain appeared to be acetylated in vivo [21] . EGFR internalization is dependent on many redundant lysine residues and involves several redundant and cooperative mechanisms [21] . Altogether, although artificial monoubiquitination of several cargos is sufficient for endocytosis, the presence of K63 polyubiquitin chains appears either critical for intracellular sorting or likely accelerates this process by increasing the avidity for Ub-binding proteins [20] , [57] , [58] , [59] , [60] , [61] . Similar observations likely applies to BRI1 Ub-mediated endocytosis. 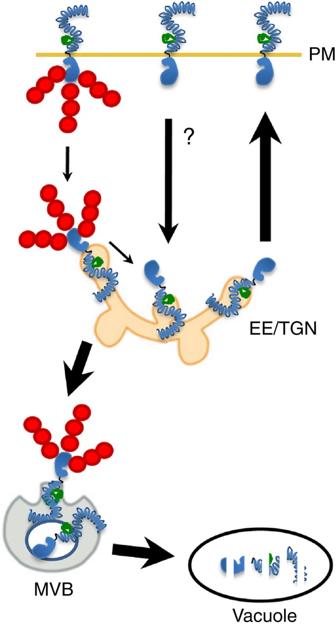Figure 7: Model for the role of ubiquitination in BRI1 endocytosis. Ubiquitination of BRI1 acts at the cell surface, redundantly with other mechanisms, to mediate BRI1 internalization. Internalized BRI1 may be deubiquitinated and recycled to the plasma membrane, or sorted into late endosomal compartments for vacuolar delivery. Ubiquitination of BRI1 is essential for proper sorting and targeting to the vacuole. Figure 7: Model for the role of ubiquitination in BRI1 endocytosis. Ubiquitination of BRI1 acts at the cell surface, redundantly with other mechanisms, to mediate BRI1 internalization. Internalized BRI1 may be deubiquitinated and recycled to the plasma membrane, or sorted into late endosomal compartments for vacuolar delivery. Ubiquitination of BRI1 is essential for proper sorting and targeting to the vacuole. Full size image Modification of BRI1 with Ub negatively regulates BRI1 function and BR signalling, as attested by the BR-hypersensitive phenotypes displayed by transgenic plants impaired in BRI1 ubiquitination. BRI1 ubiquitination is however largely independent of ligand binding, with only a transient increase in ubiquitination observed after a short-term BL treatment. This is consistent with previous observations showing that BRI1 turnover is only mildly modulated by the presence or absence of BRs [13] . BRI1 ubiquitination however required BRI1 kinase activity and the presence of its co-receptor BAK1, both mechanisms being dependent on BRs. One explanation is that in the absence of steroids, BRI1 kinase shows basal kinase activity sufficient for triggering phosphorylation of important residues for ubiquitination in BRI1 but not involved in signalling. The requirement for BAK1 is puzzling considering the BR dependency of BRI1/BAK1 interaction. However, recent evidence based on FRET-FLIM analyses indicates that significant proportion of BRI1 and BAK1 interact at the cell surface even in the absence of ligand [62] . These different observations clarify how BRI1 ubiquitination may rely on hallmarks of BR receptor complex activation, although independently of ligand perception. The ability of BRI1 to signal from endosomes has been highly debated recently [13] . The increased plasma membrane localization of BRI1 25KR , associated with enhanced BR signalling, confirms recent evidence pointing to the initiation of BR signalling at the cell surface [15] , [16] . BRI1 ubiquitination appears as a mechanism controlling the dynamics of BRI1 in the cell and thus has an impact on BR signalling, although in a BR-independent manner. Whether endogenous/exogenous cues may have an impact on BRI1 ubiquitination and thus affect BR-dependent growth will have to be investigated in the future. Plant material and constructs Wild-type (Col0), bak1-3 (ref. 63 ), bri1 T-DNA knockout [32] and the various transgenic plants generated in this study were grown at 21 °C with 16 h light/8 h dark cycles. The transgenic lines BRI1::BRI1-mCitrine, bri1 /BRI1::BRI1-mCitrine, bak1-3 /BRI1::BRI1-mCitrine and kinase-dead BRI1::BRI1 K911R -mCitrine express BRI1 under the control of its own promoter and were previously characterized [32] , [33] . mCitrine–Ub and mCitrine–Ub 7KR fusions were cloned into pDONR-P2RP3 (Invitrogen). BRI1 K866R and BRI1 25KR were cloned in pDONR221 (Invitrogen). Final destination vectors were obtained by using three-fragment recombination system using the pB7m34GW destination vectors [64] , and the entry vectors pDONR-P4P1r-BRI1prom [32] , pDONR221-BRI1 or mutated BRI1 versions, and pDONR-P2rP3-mCitrine [32] , mCitrine–Ub or mCitrine–Ub 7KR . The resulting constructs expressing BRI1 variants under the control of its own promoter were transformed into heterozygous bri1 null mutant or wild-type plants. For all constructs, more than 50 independent T1 lines were isolated and between three to six representative mono-insertion lines were selected in T2. Independent lines homozygous for the transgene when transformed in wild-type background, or for both bri1 mutation and the transgene when transformed in bri1 mutants, were selected in T3. Confocal microscopy, phenotypic analysis and protein extraction were performed on representative mono-insertional homozygous T3 lines ( Supplementary Table 1 ). Chemical treatments Inhibitors (Sigma-Aldrich) were used at the following concentrations: 2 μM ConcA (2 mM DMSO stock), 50 μM BFA (20 mM DMSO stock), 33 μM TyrA23 (50 mM DMSO stock) and 100 μM cycloheximide (CHX; 100 mM EtOH stock). BL (Chemiclones, 1 mM stock in DMSO) and BRZ (Chemiclones, 10 mM stock in DMSO) were used at concentrations indicated in the figure legends. Hypocotyl and petiole length assays Hypocotyl and petiole lengths from 15 seedlings were measured with ImageJ 1.48d on days 4 and 28, respectively. All dose–response hypocotyl elongation assays and petiole length experiments were performed in triplicates. For hypocotyl assays, imbibed seeds were stratified at 4 °C for 4 days and care was taken that seed germination occurs simultaneously between the different genotypes. Gene expression analyses Total RNA was extracted from whole plants using the RNeasy RNA extraction kit (Qiagen). SuperScript reverse transcriptase (Life Technologies) was used to synthesize cDNA from RNA. Semi-quantitative PCR using the gene-specific primers are listed in Supplementary Table 2 . Immunoprecipitation and western blot analysis Protein extraction and immunoprecipitation experiments were conducted using 12-day-old seedlings. For western blot analyses, total proteins were extracted from ~100 mg of starting material. For protein detection, the following antibodies were used: Monoclonal anti-GFP horseradish peroxidase-coupled (Miltenyi Biotech 130-091-833, 1/5,000), anti-ubiquitin P4D1 (Millipore 05-944, 1/2,500), anti K48 polyubiquitin Apu2 (Millipore 05-1,307, 1/2,000) and anti-K63 polyubiquitin Apu3 (Millipore 05-1,308, 1/2,000) [34] , anti-BRI1 (ref. 65 ) (1/2000) and anti-BES1 (ref. 12 ) 1/5000). BRI1 protein stability was determined by blocking de novo BRI1 protein synthesis with 100 μM CHX. Quantification of western blot was performed using the Densitometry plugin from Image J. Immunoprecipitation experiments were performed using 1 g of seedlings. Tissues were ground in liquid nitrogen and resuspended in 2 ml of ice-cold sucrose buffer (20 mM Tris, pH 8; 0.33 M Sucrose; 1 mM EDTA, pH 8; protease inhibitor). Samples were then centrifuged for 10 min at 5,000 × g at 4 °C. Total proteins contained in the supernatant were centrifuged at 4 °C for 45 min at 20,000 × g to pellet microsomes. The pellet was resuspended in 1 ml of immunoprecipitation buffer (50 mM Tris pH 8, 150 mM NaCl, 1% Triton X-100) using a 2-ml potter-Elvehjem homogenizer and was left on a rotating wheel for 30 min at 4 °C. Non-resuspended material was then pelleted for 10 min at 20,000 × g and 4 °C. The supernatant contained the fraction enriched in microsomal-associated proteins. Immunoprecipitations were carried out on 1 mg of microsomal proteins using the μMACS GFP isolation kit (Miltenyi Biotec). For quantification of BRI1-ubiquitinated pools, the ratio of normalized immunoprecipitation signal intensity obtained with anti-GFP and anti-Ub antibodies was determined using Image J. Immunoprecipitation and western blot analyses were performed in triplicates. Representative blots are shown in figures, and full scan blots in Supplementary Fig. 7 . Mass spectrometry Immunopurified proteins were reduced with dithiothreitol, alkylated with iodoacetamide and digested with trypsin overnight. Salts and reagents were removed by reversed phase (C-18) cartridge clean-up. The salt-free peptides were dissolved in 0.1% formic acid and subjected to ESI-MS/MS analysis on a Thermo LTQ-Orbitrap XL instrument. A capillary column (inner diameter 75 μm, packing length 10 cm of C-18 silica) with integrated spray tip was used with a 300 nl min −1 0.1% formic acid/acetonitrile gradient. Peptide precursor masses were determined with high accuracy by Fourier transform MS in the Orbitrap followed by data-dependent MS/MS of the top five precursor ions in each chromatographic time window. Data were analysed using the Mascot algorithm (Matrix Science, London, UK on a local Mascot server (version 2.1.0) and searched against the latest Swiss Protein database allowing a variable isopeptide (Gly–Gly) modification on lysine residues. Confocal microscopy Plant samples were mounted in water and viewed on Leica TCS SP2 confocal laser scanning microscopes. Images were taken at the root tip from 7-day-old plants grown in the light, or in the upper part of 4-day-old etiolated hypocotyls. For imaging mCitrine fusion proteins, the 514-nm laser line was used. Laser intensity settings were kept constant in individual sets of experiments to allow for a comparison of expression and localization of reporter proteins. Quantification of total fluorescence intensity in roots, at the plasma membrane, in intracellular compartments, in BFA bodies or in the vacuole was performed using Image J. TIRF microscopy and analysis of images Arabidopsis plantlets were grown in MS medium for 4 days in the dark to obtain etiolated hypocotyls. Hypocotyls were imaged by TIRF on a Nikon Eclipse Ti microscope equipped with a Nikon APO TIRF × 100/1.49 oil immersion objective. The excitation wavelength used was 491 nm provided by a 100-mW diode laser Toptica AOTF and emission light was collected with an emission filter Chroma ET 525/50. Time lapses were acquired during 2 min at 200-ms intervals and images were captured with a Photometrics Evolve Delta Camera using the Metamorph Software version 7.7.9.0 (Molecular Devices, LLC) and the laser power at 40%. The videos of three independent experiments were then analysed using the ImageJ 1.48d software. To better visualize the videos, the Difference of Gaussian filter and the kymographs were obtained on the treated images using the MultiKymographs plugin ( http://www.embl.de/eamnet/html/body_kymograph.html ) of ImageJ. The time of residence was determined by the duration of tracks ( n =350). To measure the density of BRI1 and BRI1 25KR at the plasma membrane, videos were treated with the Difference of Gaussian filter and the density of protein was quantified by the Find Maxima function within a region of same area using ROI manager. Each area measured was 40 × 41 pixels (0.160 μm per pixel) in size. Statistical analyses Statistical analyses were performed with the software GraphPad Prism. Physiological plant parameters (hypocotyl and petiole length), western blot and immunoprecipitation quantification used the non-parametric Mann–Whitney test (two genotypes/conditions) or the non-parametric Kruskal–Wallis (three genotypes/conditions and more) test followed by a Dunn’s or Dunnet’s post hoc test for multiple comparisons ( P <0.05). How to cite this article: Martins, S. et al . Internalization and vacuolar targeting of the brassinosteroid hormone receptor BRI1 are regulated by ubiquitination. Nat. Commun. 6:6151 doi: 10.1038/ncomms7151 (2015).